Intratumoral genome diversity parallels progression and predicts outcome in pediatric cancer Genetic differences among neoplastic cells within the same tumour have been proposed to drive cancer progression and treatment failure. Whether data on intratumoral diversity can be used to predict clinical outcome remains unclear. We here address this issue by quantifying genetic intratumoral diversity in a set of chemotherapy-treated childhood tumours. By analysis of multiple tumour samples from seven patients we demonstrate intratumoral diversity in all patients analysed after chemotherapy, typically presenting as multiple clones within a single millimetre-sized tumour sample (microdiversity). We show that microdiversity often acts as the foundation for further genome evolution in metastases. In addition, we find that microdiversity predicts poor cancer-specific survival (60%; P =0.009), independent of other risk factors, in a cohort of 44 patients with chemotherapy-treated childhood kidney cancer. Survival was 100% for patients lacking microdiversity. Thus, intratumoral genetic diversity is common in childhood cancers after chemotherapy and may be an important factor behind treatment failure. Recent studies on adult cancers have revealed extensive differences in the spectrum of somatic mutations between different parts of single primary tumours as well as between primary tumours and their metastases [1] , [2] , [3] , [4] . Such genetic intra- and intertumoral heterogeneity is clinically significant, as it confounds the analysis of biomarkers based on single tumour samples. To what extent it also has a direct impact on treatment response and progression of tumour disease has remained unclear [5] , [6] , [7] . It is also largely unknown whether the high degree of genetic variation observed in the common adult cancers [1] , [2] , [3] , [4] is also present in tumours from infants and children. To explore the landscape of somatic genome evolution in childhood cancers and its potential clinical impact, we performed high-resolution genome analyses on a group of prototypical childhood tumours, for which chemotherapy is a mandatory part of treatment. Previous studies have indicated that childhood tumours are relatively stable compared with most adult cancers, both with respect to the overall number of genome changes and the frequency of chromosomal segregation errors [8] , [9] , [10] , [11] . In contrast to these earlier studies, we now demonstrate that many chemotherapy-treated tumours in young individuals exhibit genetic diversity both within primary tumours and between primary tumours and metastases. Using in vivo xenograft models, we proceed to demonstrate that the genome profiles of metastases commonly evolve from subclones present already in the primary tumour, and that an extensive part of this evolution is driven by specific chromosome segregation defects. We finally provide evidence that intratumoral diversity per se can be used to predict outcome under current treatment protocols for the most common childhood kidney cancer, nephroblastoma. Intratumoral genome diversity in treated childhood cancers The panorama of pediatric solid malignancies outside the central nervous system is dominated by the so-called small round blue cell tumours (SRBCTs). These tumours uniformly exhibit an immature cellular phenotype, reflecting their origin from early embryonic populations such as sympathoadrenal progenitors for neuroblastoma and metanephric progenitors for nephroblastoma. While many SRBCT subtypes exhibit characteristic chromosomal rearrangements [12] , [13] , [14] , [15] , [16] , next-generation sequencing studies have shown relatively few DNA sequence mutations in childhood cancers compared with adult neoplasms [8] . The present study of intratumoral heterogeneity in SRBCTs therefore focused on genomic aberrations larger than point mutations, that is, those detectable by high-resolution genotyping arrays. The many data points given by such array-based analyses allow for precise quantification in single tumour samples of the proportion of cells harbouring each detected abnormality ( Fig. 1a,b ) [9] , [17] . Intratumoral diversity can thereby be monitored not only by comparing genomes from different locations in the same tumour (intratumoral macrodiversity) but also by dissecting genetic heterogeneity within tumour samples only a few millimetres in size (intratumoral microdiversity; Fig. 1c ). 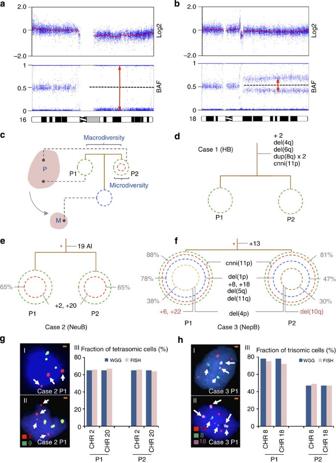Figure 1: Macro- and microdiversity in primary tumours. (a,b) Principles for microdiversity assessment exemplified by a nephroblastoma with microdiversity (T14;Supplementary Data sets 4 and 5). Relative copy number (log2) and allele ratio (BAF) for chromosomes 16 and 18 show hemizygous deletions of large parts of 16q and 18q, both resulting in loss of heterozygosity (LOH) in cells carrying the respective deletions. LOH in 100% of sampled cells would result in BAF values limited to the homozygous BAF positions 1 and 0, as observed for 16q (red arrows ina). The 18q deletion is closer to the heterozygous pattern (red arrows inb), indicating its presence in a subclone, that is, in <100% of tumour cells. (c) Diversity assessments include those comparing primary tumour and metastasis (P and M), those between samples from the primary tumour (P1 and P2; intratumoral macrodiversity), as well as diversity within each sample (intratumoral microdiversity). (d–f) Clonal tumour composition in patients with hepatoblastoma (HB), neuroblastoma (NeuB) and nephroblastoma (NepB). Each singular circle or group of concentric circles represents different tumour samples. Concentric circles of different colours depict microdiversity within a sample. Red numerals indicate aberrations not present in all biopsies from a patient and grey numerals the proportion of tumour cells where each imbalance is found. Detected imbalances include trisomy (+), deletion (del), duplication (dup) and copy number neutral imbalance (cnni). When more than five imbalances were present, the total number of allelic imbalances (AI) is given instead of detailed profiles. Red asterisks mark time points for chemotherapy. (g,h) Validation of microdiversity in Cases 2 and 3 by FISH. In Case 2, tumour cells were ascertained by trisomy 9 (Supplementary Data set 1) and interrogated for the copy numbers of chromosomes 2 and 20. Panelsg:I andg:II show tumour cells with trisomy and tetrasomy 2, respectively (arrows). In Case 3, tumour cells were ascertained by trisomy 13 and interrogated for the copy numbers of chromosomes 8 and 18. Figures h:I and h:II are examples of disomy and trisomy 8/18 (arrows). In both cases, the proportion of tumour cells with subclonal copy number alterations determined by FISH closely matched estimates by genotyping arrays (WGG;g:III andh:III). Scale bars (orange, upper right corner) correspond to 1 μm. Figure 1: Macro- and microdiversity in primary tumours. ( a , b ) Principles for microdiversity assessment exemplified by a nephroblastoma with microdiversity (T14; Supplementary Data sets 4 and 5 ). Relative copy number (log2) and allele ratio (BAF) for chromosomes 16 and 18 show hemizygous deletions of large parts of 16q and 18q, both resulting in loss of heterozygosity (LOH) in cells carrying the respective deletions. LOH in 100% of sampled cells would result in BAF values limited to the homozygous BAF positions 1 and 0, as observed for 16q (red arrows in a ). The 18q deletion is closer to the heterozygous pattern (red arrows in b ), indicating its presence in a subclone, that is, in <100% of tumour cells. ( c ) Diversity assessments include those comparing primary tumour and metastasis (P and M), those between samples from the primary tumour (P1 and P2; intratumoral macrodiversity), as well as diversity within each sample (intratumoral microdiversity). ( d – f ) Clonal tumour composition in patients with hepatoblastoma (HB), neuroblastoma (NeuB) and nephroblastoma (NepB). Each singular circle or group of concentric circles represents different tumour samples. Concentric circles of different colours depict microdiversity within a sample. Red numerals indicate aberrations not present in all biopsies from a patient and grey numerals the proportion of tumour cells where each imbalance is found. Detected imbalances include trisomy (+), deletion (del), duplication (dup) and copy number neutral imbalance (cnni). When more than five imbalances were present, the total number of allelic imbalances (AI) is given instead of detailed profiles. Red asterisks mark time points for chemotherapy. ( g , h ) Validation of microdiversity in Cases 2 and 3 by FISH. In Case 2, tumour cells were ascertained by trisomy 9 ( Supplementary Data set 1 ) and interrogated for the copy numbers of chromosomes 2 and 20. Panels g :I and g :II show tumour cells with trisomy and tetrasomy 2, respectively (arrows). In Case 3, tumour cells were ascertained by trisomy 13 and interrogated for the copy numbers of chromosomes 8 and 18. Figures h:I and h:II are examples of disomy and trisomy 8/18 (arrows). In both cases, the proportion of tumour cells with subclonal copy number alterations determined by FISH closely matched estimates by genotyping arrays (WGG; g :III and h :III). Scale bars (orange, upper right corner) correspond to 1 μm. Full size image We first performed high-resolution whole-genome genotyping single-nucleotide polymorphism (SNP) array analysis of seven SRBCT patients from whom multiple tumour samples had been collected either from the same tumour or from both primary and secondary tumours/metastases ( Figs 1d–f and 2a–d ; Table 1 ; Supplementary Data set 1 ). Microdiversity was detected in five of the seven patients (Cases 2–5 and 7; Figs 1e–f and 2a,b,d ; Supplementary Fig. 1a,b ), as demonstrated by genomic imbalances present in different proportions of tumour cells in single samples (≈3 mm in size). In all patients sampled after chemotherapy microdiversity was present. In contrast, no microdiversity was found in Cases 1 and 6, from which all samples were obtained before chemotherapy. Macrodiversity in the primary tumour could be assessed in cases 1–4, from whom two or more biopsies (>2 cm apart) were analysed ( Figs 1d–f and 2a ). Case 1 exhibited neither micro- nor macrodiversity. In Case 2, both samples from the primary tumour showed microdiversity with a highly similar clonal composition. Cases 3 and 4 exhibited a clear connection between micro- and macrodiversity. In Case 3, the only differences between the two primary tumour samples P1 and P2 were found in subclones making out 38 and 30% of tumour cells, respectively ( Fig. 1f ). In Case 4, a large neuroblastoma of the abdomen was observed from which samples were taken at a distance of 10 cm apart; the genome profile of one sample (P2) clearly derived from a trisomy 7-bearing subclone found in the other biopsy (P1; Fig. 2a ). Hence, intratumoral diversity appeared to be a common feature of chemotherapy-treated childhood tumours, with macrodiversity often resulting from shifting landscapes of microdiversity. 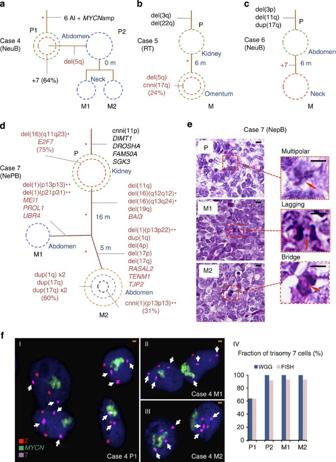Figure 2: Genome profiles of primary versus secondary tumours. Tumour types, allelic imbalances, subclones and chemotherapy treatment are annotated as inFig. 1. Evolutionary ideograms are used to display relationships between subclones in the primary tumours (P) and the genome profiles of secondary tumours (metastases, M). Connecting lines are drawn from subclonal layers giving rise to secondary tumours. (a–d) Clonal composition of patients with NeuB, renal rhabdoid tumour (RT) and NepB are depicted. Time between samples is given in months (m). Case 7 was also analysed by exome sequencing. Here single-nucleotide variants and small indels are indicated by gene symbols (Supplementary Data set 2). The 16q deletions in the primary tumour (P) and the first metastasis (M1) have different breakpoints but involved partly the same chromosome segments (Supplementary Data set 1), indicating convergent evolution (single diamond symbols). There was also evidence of convergent evolution in the form of different loss of heterozygosity events in 1p, covering overlapping genome segments in M1 and M2 (double diamond symbols). (e) While the primary kidney tumour in Case 7 showed mixed-type intermediate risk histology, M1 and M2 showed identical morphology dominated by small round blue blastic cells (scale bars=10 μm). Mitotic segregation errors were found in tissue sections in both primary and recurrent tumours, as exemplified by magnified images (red arrows; scale bars=10 μm). (f) Validation of microdiversity in Case 4 by FISH. Tumour cells were ascertained by the presence ofMYCNamplification. Both FISH and WGG arrays (f:IV) showed a mix of cells with disomy and trisomy 7 in P1 (f:I; arrows point to centromere probe 7), while the other three samples contained >90% trisomic cells (f:II andf:III). Scale bars (orange, upper right corner) correspond to 1 μm. Figure 2: Genome profiles of primary versus secondary tumours. Tumour types, allelic imbalances, subclones and chemotherapy treatment are annotated as in Fig. 1 . Evolutionary ideograms are used to display relationships between subclones in the primary tumours (P) and the genome profiles of secondary tumours (metastases, M). Connecting lines are drawn from subclonal layers giving rise to secondary tumours. ( a – d ) Clonal composition of patients with NeuB, renal rhabdoid tumour (RT) and NepB are depicted. Time between samples is given in months (m). Case 7 was also analysed by exome sequencing. Here single-nucleotide variants and small indels are indicated by gene symbols ( Supplementary Data set 2 ). The 16q deletions in the primary tumour (P) and the first metastasis (M1) have different breakpoints but involved partly the same chromosome segments ( Supplementary Data set 1 ), indicating convergent evolution (single diamond symbols). There was also evidence of convergent evolution in the form of different loss of heterozygosity events in 1p, covering overlapping genome segments in M1 and M2 (double diamond symbols). ( e ) While the primary kidney tumour in Case 7 showed mixed-type intermediate risk histology, M1 and M2 showed identical morphology dominated by small round blue blastic cells (scale bars=10 μm). Mitotic segregation errors were found in tissue sections in both primary and recurrent tumours, as exemplified by magnified images (red arrows; scale bars=10 μm). ( f ) Validation of microdiversity in Case 4 by FISH. Tumour cells were ascertained by the presence of MYCN amplification. Both FISH and WGG arrays ( f :IV) showed a mix of cells with disomy and trisomy 7 in P1 ( f :I; arrows point to centromere probe 7), while the other three samples contained >90% trisomic cells ( f :II and f :III). Scale bars (orange, upper right corner) correspond to 1 μm. Full size image Table 1 Characteristics of Cases 1–7. Full size table To validate the precision of microdiversity estimates made by genome arrays, the intratumoral prevalence of selected genomic imbalances was also determined by fluorescence in situ hybridization (FISH) on tumour touch preparations and formalin-fixed tissue sections from all seven cases (Cases 2–4 in Figs 1g,h and 2f ; Cases 1, 4 and 5–7 in Supplementary Fig. 2 ). Overall, there was excellent concordance between genome arrays and FISH, with a median difference in clone size estimates of 2% and a maximum difference of 8% (17 validation experiments in total). In all cases subjected to validation, FISH analysis could confirm the presence of microdiversity that had been detected by genome array. Branching and convergent evolution in metastases Differences between primary and secondary (metastatic) tumours could be analysed in four cases (Cases 4–7 in Fig. 2a–d ). All comparisons showed that additional mutations had been acquired in metastases compared with the simplest set of aberrations found in the primary tumour. Two of these patients (Cases 4 and 7) showed a clear connection between microdiversity in the primary tumour and the genome profile of metastases. In Case 4, a specific subclone had expanded within the primary tumour and gave rise to the genome profile of the metastasis ( Fig. 2a ). In Case 7, a subclone within the primary tumour in the kidney was the origin of two subsequent metastases in the abdomen after chemotherapy ( Fig. 2d ). To illustrate clonal evolution further in this patient, whole-exome sequencing was performed. In the primary tumour, this revealed three somatic missense mutations and two somatic deletions of two to three bases that were validated by deep resequencing ( Supplementary Data set 2 ). Four of these alterations, including a heterozygous mutation of the key micro-RNA regulator DROSHA , were also detected in the two metastases (M1 and M2). Apart from mutations present in the primary tumour, the metastases were related through four deletions and a BAI3 mutation. The only mutation scored as subclonal was the E2F7 mutation in the primary tumour (P), with read numbers giving an estimated prevalence of 75%, similar to the subclonal 16q deletion. M1 and M2 also showed multiple, unique large-scale genomic imbalances and sequence mutations, as well as microdiversity in M2. Despite these differences in tumour genomes, the metastases showed a remarkably similar morphology, dominated by monomorphic blastic cells ( Fig. 2e ). Also, there was evidence of convergent evolution in the form of different mechanisms in different samples giving rise to similar allelic imbalances, including loss of heterozygosity events in 1p and 16q (see legend to Fig. 2d for details). Chromosomal instability drives genome evolution Considering that only one or two samples were acquired from each primary tumour in Cases 4–7, it could not be excluded that seemingly novel aberrations in secondary tumours reflected expansion of subclones already present in their respective disease primary lesions. To monitor further the relationship between genome diversity in primary and secondary SRBCT populations, we constructed a xenograft-based model of aggressive metastatic disease with secondary tumour evolution. This was carried out by comparing in vitro genome profiles of three cell lines (CL1–3) established in long-term culture from two nephroblastomas and one neuroblastoma ( Supplementary Data set 3 ), to NOD SCID gamma (NSG) mouse retroperitoneal xenograft tumours derived from 200,000 cells from twin cultures of CL1–3 ( Fig. 3a–c ). This revealed a remarkable difference in the capacity to evolve novel genome profiles in secondary tumours among the cell lines. Only one novel aberration was found in CL1 xenografts, an intermediate number in CL2 xenografts and a very high number in CL3 xenografts. Analysis of ana-telophase figures in CL1–3 cells obtained before injection, including the frequency of lagging chromosomes, anaphase bridging and multipolar cell divisions showed that the frequency of such errors increased in proportion with each cell line’s capacity to form novel aberrations in secondary tumours ( Fig. 3d–f ). The same type of mitotic defects was also found in the primary SRBCTs from which samples could be obtained (Cases 1–4, 6–7; tissue not available for Case 5; Fig. 2e , right panel; Supplementary Figs 3,4 ). Precise quantification of segregation errors was not possible because of scarcity of mitoses in tumour sections, but these findings ruled out segregation errors as in vitro artifacts in SRBCT cells. 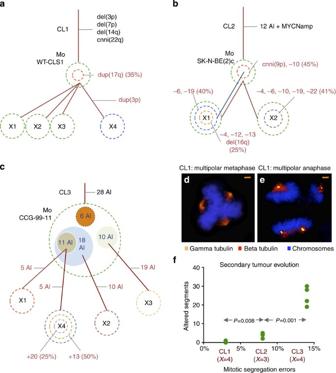Figure 3:In vivomodelling of secondary tumour formation. Genome profiles ofin vitromother populations (Mo) of the SRBCT cell lines WT-CLS1 (CL1), SK-N-BE(2)c (CL2) and CCG-99-11 (CL3) were compared with genotypes of secondary tumours/xenografts (X) formed by cell line injection into NSG mice. One secondary tumour formed at each injection site. (a–c) Evolutionary relationships between Mo and X for CL1-3 are depicted by ideograms as inFig. 2. Connecting lines are drawn from subclonal layers, giving rise to secondary tumours. In CL2, two of the tumour cell populations in the mother culture contributed to the different subclones in the secondary tumour X1 (blue and brown lines). In CL3, several aberrations in the genome profiles of xenografts could be traced back to subclones in the mother population, allowing further dissection of its subclonal composition. The number of allelic imbalances characteristic of each subclone in CL3 Mo are shown in blue type (Supplementary Data set 4). X1 and X4 originated from a common subclone with 11 unique allelic imbalances, which had formed from a clone with 18 unique imbalances, also giving rise to X2. X3 derived from another subclone with 10 unique imbalances. Six additional subclonal aberrations unique to the mother culture (orange circle) were also detected. (d,e) Representative images from CL1 show multipolar metaphase (d) and anaphase (e) cells. Scale bars (orange, upper right corner) correspond to 1 μm). (f) The frequency of mitotic segregation errors differed between cell lines and increased together with the number of novel aberrations/altered segments observed by comparing mother cultures and xenografts.Pvalues were obtained by Student’st-test. Figure 3: In vivo modelling of secondary tumour formation. Genome profiles of in vitro mother populations (Mo) of the SRBCT cell lines WT-CLS1 (CL1), SK-N-BE(2)c (CL2) and CCG-99-11 (CL3) were compared with genotypes of secondary tumours/xenografts (X) formed by cell line injection into NSG mice. One secondary tumour formed at each injection site. ( a – c ) Evolutionary relationships between Mo and X for CL1-3 are depicted by ideograms as in Fig. 2 . Connecting lines are drawn from subclonal layers, giving rise to secondary tumours. In CL2, two of the tumour cell populations in the mother culture contributed to the different subclones in the secondary tumour X1 (blue and brown lines). In CL3, several aberrations in the genome profiles of xenografts could be traced back to subclones in the mother population, allowing further dissection of its subclonal composition. The number of allelic imbalances characteristic of each subclone in CL3 Mo are shown in blue type ( Supplementary Data set 4 ). X1 and X4 originated from a common subclone with 11 unique allelic imbalances, which had formed from a clone with 18 unique imbalances, also giving rise to X2. X3 derived from another subclone with 10 unique imbalances. Six additional subclonal aberrations unique to the mother culture (orange circle) were also detected. ( d , e ) Representative images from CL1 show multipolar metaphase ( d ) and anaphase ( e ) cells. Scale bars (orange, upper right corner) correspond to 1 μm). ( f ) The frequency of mitotic segregation errors differed between cell lines and increased together with the number of novel aberrations/altered segments observed by comparing mother cultures and xenografts. P values were obtained by Student’s t -test. Full size image The model also provided detailed information regarding the relationship between genome profiles of secondary/xenograft tumours and microdiversity in their populations of origin. The chromosomally stable CL1 contained few novel aberrations in its xenografts. In contrast, several aberrations not detected in all cells of the original cell line were found in CL2 X1 and X2, giving each a distinct profile ( Fig. 3b ). At least one of the X1 subclones derived from a clone already present in the primary cell population as they both shared a unique structural aberration in 9p. Similarly, the four CL3 xenografts contained a total number of 78 allelic imbalances that were not present in all cells in the mother cell line. Of these, 50% (39/78) could be traced back to a common subclonal origin in the mother line, either because they were detected in a minority cell population in the mother line or because of specific genomic breakpoints that were identical in more than one xenograft tumour ( Fig. 3c ; Supplementary Data set 4 ). Although care should be taken in projecting data from xenografted cell lines to a human in vivo context, the results from CL2 and CL3 supported indications from the primary tumour set that significant features of SRBCT metastasis genomes derive from subclones that evolved extensively already in the primary tumour, as shown previously for several adult cancers [4] , [18] , [19] , [20] . The xenograft models also provided as strong indication that the rate of chromosome segregation errors in the founder cell population may determine the extent of genome evolution over time. Microdiversity predicts outcome after chemotherapy Based on the indications that genetic diversity in primary tumours predisposed to further genome evolution in SRBCTs, we hypothesized that the presence of microdiversity in primary tumour samples could be used as a biomarker for disease progression. To test our theory, we used follow-up data from a cohort of 44 nephroblastomas treated within the recently closed SIOP2001 Nephroblastoma Trial and Study ( Supplementary Data set 5 ). This protocol consists of both pre- and postoperative chemotherapy [21] , and all biopsies were obtained from tumour-nephrectomy specimens obtained ~7 days after the last chemotherapy cycle. Our cohort was representative of nephroblastoma with regard to the panorama of genomic imbalances and had survival statistics that stratified according to established clinicopathological parameters ( Supplementary Figs 5 and 6a–c ) [22] , [23] . High-resolution genome array analysis showed microdiversity in 45% (20/44) of the tumours ( Supplementary Fig. 1c–h ; Supplementary Data sets 5 and 6 ). There was no significant difference in age between patients with and without microdiversity ( P =0.12; Student’s t -test). Microdiversity was more prevalent in tumours with high risk compared with low- or intermediate risk histology, in high- compared with low-stage disease, as well as in tumours of patients dead of disease compared with long-term survivors ( Fig. 4a,b ). Tumours with microdiversity also showed more allelic imbalances than those without microdiversity ( Fig. 4c,d ). 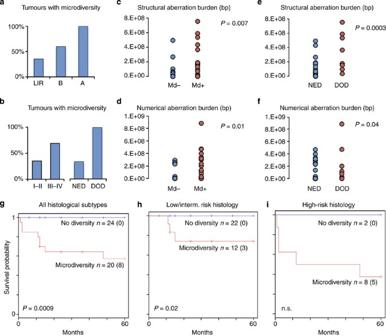Figure 4: Clinical correlations to microdiversity in primary tumours. (a,b) Graphic presentation of the fraction of cases with microdiversity among histological subtypes of nephroblastoma (LIR, low- and intermediate risk; B, blastemal high risk; A, diffuse anaplastic high risk) and in tumour disease of various stages (I–II, confined to the kidney; III–IV, extrarenal spread), as well as in patients who died of disease (DOD) compared with those having no evidence of disease (NED) after follow-up (mean follow-up time is 46 months; range 1–144 months). (c,d) Tumours with microdiversity (Md+) also showed more allelic imbalances affecting segments of chromosomes (structural aberrations) and whole chromosomes (numerical aberrations). The allelic imbalance burden per tumour reflects the total sum of genomic regions affected by imbalance;Pvalues from Student’st-test. (e,f) There was also a difference in the number of imbalances among tumours from patients with different outcomes, but with large variation within the groups. (g) Tumours with microdiversity were associated with a lower cancer-specific survival than those without diversity in the entire cohort. (h) A difference in cancer-specific survival was also observed in the large subgroup (33/44 patients) with low-intermediate risk histology. (i) There was also a trend of a similar impact on cancer-specific survival for tumours with high-risk histology;Pvalues were obtained by the log-rank test. Figure 4: Clinical correlations to microdiversity in primary tumours. ( a , b ) Graphic presentation of the fraction of cases with microdiversity among histological subtypes of nephroblastoma (LIR, low- and intermediate risk; B, blastemal high risk; A, diffuse anaplastic high risk) and in tumour disease of various stages (I–II, confined to the kidney; III–IV, extrarenal spread), as well as in patients who died of disease (DOD) compared with those having no evidence of disease (NED) after follow-up (mean follow-up time is 46 months; range 1–144 months). ( c , d ) Tumours with microdiversity (Md+) also showed more allelic imbalances affecting segments of chromosomes (structural aberrations) and whole chromosomes (numerical aberrations). The allelic imbalance burden per tumour reflects the total sum of genomic regions affected by imbalance; P values from Student’s t -test. ( e , f ) There was also a difference in the number of imbalances among tumours from patients with different outcomes, but with large variation within the groups. ( g ) Tumours with microdiversity were associated with a lower cancer-specific survival than those without diversity in the entire cohort. ( h ) A difference in cancer-specific survival was also observed in the large subgroup (33/44 patients) with low-intermediate risk histology. ( i ) There was also a trend of a similar impact on cancer-specific survival for tumours with high-risk histology; P values were obtained by the log-rank test. Full size image Although the total burden of rearrangements was higher in high-risk morphology tumours and in tumours of patients who later died of disease, the substantial variation in aberration burden within these clinical groups prevented a clear-cut risk stratification within most subgroups based on the number of imbalances ( Fig. 4e,f and Supplementary Fig. 6e–h ). For the entire nephroblastoma cohort, we also calculated the weighted genome instability index (wGII), previously used to classify colorectal cancers into cases with (CIN+) and without (CIN−) chromosomal instability based on genome array data [24] . CIN+ cases (wGII>0.2) were confined to the group of tumours with microdiversity (5/20 cases; Supplementary Fig. 7 ). Although patients who died of disease were significantly over-represented in the CIN+ group (4/5 versus 4/39; P =0.0024; Fisher’s exact test), deaths were equally distributed between the CIN+ and CIN− groups (four deaths in each) and also patients with very low wGII died of disease. Taken together, wGII and parameters derived from the sum of genomic aberrations were suboptimal for risk stratification. In contrast, the absence and presence of microdiversity appeared to be a viable parameter for risk stratification in our cohort. The survival rate was 100% for patients without tumour microdiversity, irrespective of stage and histological subgroup. Microdiversity significantly predicted cancer-specific and event-free survival both in the entire patient cohort and within the largest histopathological risk group ( Fig. 4g,h and Supplementary Fig. 6i,j ), where it was in fact a better predictor than stage (compare Fig. 4h with Supplementary Fig. 6d ). There were also trends of inferior outcome for tumours with microdiversity within the small subset of high-risk histology tumours and for patients of similar stage ( Fig. 4i and Supplementary Fig. 6k,l ). Multivariate analysis was performed using a Cox proportional hazards model including tumour stage, histological risk group, tumour microdiversity (quantified as the number of subclonal imbalances) and the total number of non-subclonal genomic imbalances. This showed microdiversity (the number of subclonal aberrations) to be the only independent predictor of cancer death in our cohort (hazard ratio 1.06 per subclonal aberration; 95% confidence interval 1.0006–1.12; Wald test P =0.005). The low number of events precluded a more extensive multivariate analysis. The panorama of genetic diversity in childhood cancers has not been extensively explored. Recent next-generation sequencing, based on single samples from each tumour, has shown relatively few mutations and chromosome rearrangements in solid childhood malignancies [25] , [26] , [27] , [28] . This has led to the notion that cancer genomes in children are relatively stable [8] , which has been supported by findings of a high level of chromosome segregation errors limited to very aggressive childhood cancer subtypes [11] . In contrast, prototypical adult malignancies such as adenocarcinomas and soft tissue sarcomas commonly exhibit a high frequency of chromosomal instability ascertained by mitotic segregation errors [29] , [30] . The present study of clonal evolution under chemotherapy does not support the notion of childhood cancers being overall genetically stable. Our data show that intratumoral diversity is common in chemotherapy-treated primary childhood cancers and that such diversity can provide a substrate for further genome evolution in metastases. Intratumoral diversity in the form of microdiversity could be found after chemotherapy irrespective of histology as evidenced by its presence in at least three different entities, that is, neuroblastoma, nephroblastoma and rhabdoid tumour. This is interesting, as these three tumour types exhibit very different patterns of chromosomal imbalances. Neuroblastomas often have complex structural or numerical aberrations, while nephroblastomas and rhabdoid tumours typically have karyotypes of low complexity. Our xenograft models indicated that fundamental chromosome segregation defects was a likely contributor to metastatic genome evolution. Our analysis of multiple tumour samples from the same patients failed to provide a uniform view of how childhood cancer genomes evolve over space and time. Similar to the scenario in adult cancers, there was a wide variation in the extent to which different tumour samples showed genetic variability [31] . It is noteworthy that some tumours (Cases 2 and 3; Fig. 1e,f ) exhibited a remarkable similarity in the clonal composition found in different tumour areas, indicating that the panorama of genetic diversity can be maintained over relatively large distances (>2 cm). This could suggest that tumour growth in some instances benefit from maintaining a balance between subpopulations of neoplastic cells with different genotypes. Whether this is a sign of tumour cell interdependence for optimal growth remains to be explored [32] . On the other hand, there was also evidence of clonal evolution followed by expansion of a subclone up to a point where genetic diversity was largely eliminated (Case 4; Fig. 2a ). This may reflect a subclone’s acquisition of a genotype with considerably higher fitness than its founder population. In the context of chemotherapy treatment, it is tempting to suggest chemotherapy resistance to be one factor behind such clonal expansions, leading to the extinction of the founder genotype. While the majority of genomic imbalances confined to subclones were low-frequency aberrations in their respective tumour subtypes according to previous studies, there were indeed also examples of highly recurrent, potential drivers, emerging as part of microdiversity landscapes. In nephroblastomas these included copy number neutral imbalance of 11p and trisomy 8 (Case 2), as well as 1q gain and 1p/16q loss (Case 7)—all of which are highly prevalent and characteristic abnormalities in this tumour type [15] . Metastases overall showed divergent genome profiles compared with the least complex clone in their respective primary tumours, indicating branching clonal evolution (Cases 4–7 and CL1–C3; Figs 2 and 3 ). However, there was also evidence of convergent evolution in metastases in Case 7 ( Fig. 2d ). In this case, independent mutation events, with different chromosomal breakpoints, led to repeated occurrence of both 1p and 16q loss of heterozygosity over time. This is particularly interesting as both these aberrations are strongly associated with high-risk morphology and poor outcome [22] , [23] , [33] . Genome profiles in metastases frequently derived from subclones that were part of a microdiversity landscape. This was best illustrated by our xenograft models of secondary tumour evolution, as this experimental design allowed genetic profiling of the entire founder cell population, in contrast to Cases 4–7, where only selected parts of the primary tumours could be assessed. In summary, our attempts to profile tumour genome development over space and time in vivo , showed that branching evolution appears to be the norm in childhood cancers under treatment, that this scenario can be modelled and related to chromosomal instability by xenograft models in animals and that microdiversity appears to provide a fertile substrate for further genome evolution. We also found that microdiversity per se could serve as a potential predictive biomarker. Using microdiversity to obtain actionable clinical information is a novel concept. It provides a stark contrast to current strategies for biomarker evaluation, with mutation status, genome profile or protein expression typically being evaluated in merely a single tumour sample—resting on the assumption that tumours are biologically homogeneous [5] . Microdiversity would be a particularly attractive clinical marker as it is a parameter possible to quantify using standard genome arrays and relatively simple bioinformatic operations [17] . The fact that we found a potential prognostic value of microdiversity in preoperatively treated nephroblastoma may be of particular interest because there is currently no standard molecular prognosticator for the many children worldwide treated for nephroblastoma under protocols with mandatory preoperative chemotherapy. However, it should be stressed that our nephroblastoma cohort is small and that future, preferably prospective, studies are needed to validate further the clinical utility of microdiversity quantifications in childhood cancer. It should also be taken into account that the absence or presence of microdiversity may in some cases vary between different parts of a tumour (Case 4; Fig. 2a ), which may confound clinical risk assessment. Furthermore, it is unlikely that the prognostic value of microdiversity is equally strong in all SRBCTs as this group consists of biologically diverse tumour types with a wide variety of clinical predictors. Nevertheless, the present study shows unambiguously that intratumoral genome diversity in treated childhood cancers is common and sometimes extensive. Its role as a foundation for tumour cell evolution and as a confounding factor in biomarker studies based on single tumour samples should not be disregarded in children with cancer. Patients and tumour material The present study was approved by the Regional Ethics Board of Southern Sweden (permit nos 119–2003 and 289–2011). Written informed consent for genomic analyses was obtained from the patients’ parents or guardians. Tumour tissue was collected as a part of clinical diagnostic procedures. Material for genomics was frozen immediately after arrival at the pathology laboratory and stored at −80 °C until DNA extraction. Biopsies from the same tumour were taken at least 2 cm apart. DNA was extracted from tumour tissue volumes of ~3 × 3 × 3 mm. Samples from cases 1–7 were obtained during 2001–2004. Cases 1–3, 5 and 7 initially presented with localized disease, the remaining cases with disseminated tumour. Nephroblastoma samples from post-chemotherapy tumour-nephrectomies were obtained under the SIOP2001 study, from a consecutive series of 58 patients, from which tumours without allelic imbalances by SNP array (14 patients) were excluded, as the tissue representativity was questionable. The remaining patient material was still overall representative of nephroblastoma with a slight female over-representation (1.2:1) and a mean age of 3.7 years. The mean follow-up time was 46 months. The preoperative chemotherapy was according to the SIOP2001 Nephroblastoma Trial and Study and consisted of 4 and 6 weeks of vincristine (V) and actinomycin D (A) for localized and metastatic disease, respectively, with addition of doxorubicin (D) for the latter. Surgery and sampling for genomics occurred per protocol 7 days after the finalization of preoperative chemotherapy. Local stage and histological risk classification at surgery determined the post-surgical regimen. Intermediate risk implied AV regimens of 4–27 weeks with the addition of radiotherapy if stage III. High-risk stage I implied AVD for 27 weeks and for stages II–III cyclophosphamide, etoposide, doxorubicin and carboplatin for 34 weeks including irradiation. Whole-genome genotyping by SNP arrays Tumour DNA was extracted by the DNeasy Blood & Tissue Kit (Qiagen, Valencia, CA) according to the manufacturer’s description. DNA was hybridized to HumanCNV370-Duo/Quad Genotyping BeadChips, 1 M Genotyping BeadChip HumanOmni1-Quad (Illumina Inc., San Diego, CA), or Affymetrix Cytoscan HD (Affymetrix, Santa Clara, CA). Aberration calling from Illumina chips was as previously described [33] . The Chromosome Analysis Suite (ChAS, Affymetrix) Software was used to analyse Affymetrix Cytoscan HD data, followed by bioinformatic analysis with TAPS [34] . Copy number aberrations were considered if 10 or more consecutive markers/SNPs qualified as loss or gain. Constitutional copy number variants were omitted based on manual comparison against the Database of Genomic Variants ( http://dgv.tcag.ca ). Segmented raw data from SNP arrays are presented in Supplementary Data sets 1, 3 and 6 . Quantification of microdiversity Cancer cell content in tumour samples from Cases 1–7 was assayed by SNP array as specified below and also validated histologically in parallel haematoxylin–eosin-stained tissue sections. The cancer cell fraction ranged from 60 to 99%, well in agreement with clearly deviant SNP array profiles, which fulfilled local criteria for clinical analysis ( Supplementary Figs 8–11 ). The method for estimating the proportion of cells containing a certain allelic imbalance from Illumina arrays has previously been validated by us and others [9] , [17] , [35] , [36] . In brief, the fraction of cells within single tumour samples that harboured each detected allelic imbalance was calculated using mirrored B-allele frequency (mBAF) values from the BAF-segmentation algorithm for Illumina arrays [35] . This method filters out noninformative homozygous SNPs and provides segments specified by genomic position, log2 value and the mBAF value. In a diploid background the mBAF values were used to directly calculate the estimated tumour cell content of each allelic imbalance using the formula: Here f is the fraction of cells in a sample containing a certain allelic imbalance, and B and A are the absolute numbers of the two alleles for heterozygous loci. When nondiploid, calculations were normalized for tumour cell ploidy as obtained by SNP array assessment, or cytogenetic analyses in cases where SNP array interpretation was ambiguous with respect to ploidy. The bioinformatic tool TAPS [34] was used for Affymetrix arrays to estimate absolute allele-specific copy numbers and identify genomic regions with copy number heterogeneity and the most likely composition of copy numbers behind each such observation, as described [34] . The median intensity ratio (2 log ratio ; or BAF in case of copy-neutral heterogeneity) of an identified region was used to calculate relative prevalence of each copy number in the composition, using genomic segments with the involved copy numbers in all tumour cells as reference points. Tumour DNA fraction DNAfrac Tum was estimated from the observed difference in intensity ratio associated with one more or less copy in all tumour cells Δ obs , relative to the expected Δ exp fom 100% tumour cells (Formula 1). Δ exp is based on the average ploidy of the tumour cells Ploidy Tum and the difference in intensity ratio Δ X associated with one more or less copy in a normal diploid genome for the particular microarray (Formula 2). Tumour cell fraction Cellfrac Tum was then calculated by compensating for any aberrance in DNA content per tumour cell Ploidy Tum relative to that of normal cells Ploidy Norm =2 (Formulae 3 and 4). Genome segments of <0.2 Mb were excluded from microdiversity analysis to ensure reliable prevalence estimates. Sex chromosomes were not included in the analyses to avoid somatic mosaicism as a confounding factor. Whole-exome sequencing Exome-sequencing libraries from Case 7 were prepared from genomic DNA from the primary tumour, the two metastases and blood using the Truseq Exome enrichment kit (Illumina) according to the manufacturer’s instructions. The libraries were subjected to paired end 100 bp sequencing on a HiScanSQ (Illumina). Reads were aligned to the human reference genome (hg19) using bwa 0.5.9 (ref. 37 ), and PCR duplicates within the alignments were identified using Picard 1.57 ( http://picard.sourceforge.net ). Reads around insertions and deletions (indels) were realigned and base-calling quality scores were recalculated using IndelRealigner, CountCovariates and TableRecalibration from the Genome Analysis Toolkit version 1.3–24 (ref. 38 ) Somatic single-nucleotide variants were identified from the alignments using SomaticCall version r39433 ( http://www.broadinstitute.org/science/programs/ genome-biology/computational-rd/somaticcall-manual). Somatic indels were identified using SomaticIndelDetector from the Genome Analysis Toolkit. Putative nonsynonymous somatic variants were verified by targeted exon sequencing. A custom SureSelect kit (Agilent Technologies, Santa Clara, CA) was used to capture the exons of interest flanked by 25 bps together with 5′ and 3′ untranslated repeats. DNA was sheared by sonication with the Covaris S2 instrument (Covaris Inc., Woburn, MA). Fragment libraries were created from the sheared samples using the AB Library Builder System (Life Technologies, Grand Island, NY) and target enrichment was performed according to the manufacturer’s protocols. Target capture was conducted by hybridizing the DNA libraries with biotinylated RNA baits for 24 h followed by extraction using streptavidin-coated magnetic beads. Captured DNA was then amplified followed by emulsion PCR using the EZ Bead System (Life Technologies) and sequenced on the SOLiD5500W system. Coverage was in the range of 700–2,000 × . Alignment of reads to the human reference sequence (hg19) and variant calling was performed using v2.1 of the LifeScope software. ANNOVAR ( http://www.openbioinformatics.org/annovar/ ) was used to annotate genes and amino-acid changes and to filter the data against databases of known constitutional variants (dbSNP 130, 1000 genomes2012, esp6500) [39] . Putative variants covered by less than 10 reads, together with polymorphisms present in the blood of Case 7 were removed from the study. Reads indicating potential mutations were visually inspected with the Integrative genomics viewer ( http://www.broadinstitute.org/igv/ ) [40] , [41] , and variants covered by reads with poor quality were discarded. Resulting filtered raw data on mutations are present in Supplementary Data set 2 . Fluorescence in situ hydridization FISH validation experiments were performed on touch preparations from frozen tissue samples from Cases 1–7 as well as on formalin-fixed paraffin-embedded tissue sections from Case 4. Cases 1 and 7 were estimated by genome arrays and cytomorphology to contain >95% tumour cells making additional probes for the ascertainment of tumour cell identity redundant. To ascertain the neoplastic identity of cells in the remaining cases, the following markers were used, based on findings of whole-genome genotyping array data: trisomy 9 in Case 2; trisomy 13 in Case 3; MYCN amplification in Case 4; 22q deletion in Case 5; and 17q duplication in Case 6. In these cases, analyses were limited to cells positive for these markers. Centromere probes and probes for 2p24 ( MYCN ), 8q ( MYC ), 13q ( RB1 ), 17q and 22q ( BCR/ABL1 ) were purchased from Abbott Molecular (Abbott Laboratories, Abbott Park, IL), while the 5q probe used in Case 5 was prepared from the BAC clone RP11-90C21 (BACPAC Resources Center, Children’s Hospital Oakland Research Institute, Oakland, CA). Touch preparations, probe manufacturing, hybridization, stringency washing and analyses were performed as previously described [42] . Tissue sections were subjected to hybridization after antigen retrieval and 10 min of treatment by 0.01% pepsin as described [9] . At least 100 nonoverlapping nuclei were analysed in each FISH experiment. Animal xenograft models All animal procedures followed the guidelines set by the Malmö-Lund Ethical Committee for the use of laboratory animals and were conducted in accordance with the European Union directive on the subject of animal rights (M331-11). The established nephroblastoma cell lines WT-CLS1 and CCG-99-11, and the neuroblastoma cell line SK-N-BE(2)c were cultured in standard medium supplemented with 10% fetal bovine serum and 1% Penicillin Streptomycin. At 4–6 weeks of age, female NSG mice (Charles River Laboratories, Wilmington, MA) were anaesthetized using 2–3% isofluorane inhalation and Temgesic was administered subcutaneously. An incision was made to access the retroperitoneal space on the left side and 2 × 10 5 tumour cells in 30 μl PBS were injected into the kidney (WT-CLS1 and CCG-99-11) or adrenal gland (SK-N-BE(2)c). Mice were killed immediately when they exhibited general symptoms of tumour growth, that is, 89–92 days for WT-CLS1, 37–41 days for CCG-99-11 and 31 days for SK-N-BE(2)c. Xenograft tumours that formed at the injection sites were snap-frozen and stored in −80 °C before genomic assays. Quantification of mitotic segregation errors The frequency of chromosome segregation errors in CL1–3 cell cultures was obtained as previously described [43] , using gamma and beta tubulin as markers for centrosomes and the mitotic spindle microtubules, respectively. Segregation errors were scored in a minimum of 30 ana-telophase cells and classified into multipolar spindles, chromatin bridges and lagging chromosomes/chromatids according to established parameters [44] . Because all three classes of segregation errors correlated strongly to each other in each cell line, the percentages of each type of error were summarized to obtain the final score of mitotic segregation errors. Histological slides were scanned at × 40 magnification on an Aperio AT2 Slide Scanner and analysed using Aperio ImageScope (Leica Biosystems, Kista, Sweden). Survival statistics Factors influencing survival in the nephroblastoma cohort were analysed using R 3.1.1, using the survival package and the survfit , survdiff and coxph functions. The wGII was calculated as described in ref. 24 . Briefly, for each autosome the number of bases deviating from the modal number (2 n ) was added together using the segment data in Supplementary Data set 6 , and this sum was normalized to the size of the chromosome in question. For each sample, the mean for all chromosomes were calculated, and this was used as the sample wGII. How to cite this article: Mengelbier, L. H. et al . Intratumoral genome diversity parallels progression and predicts outcome in pediatric cancer. Nat. Commun. 6:6125 doi: 10.1038/ncomms7125 (2015).